Tablet-level origin of toughening in abalone shells and translation to synthetic composite materials Nacre, the iridescent material in seashells, is one of many natural materials employing hierarchical structures to achieve high strength and toughness from relatively weak constituents. Incorporating these structures into composites is appealing as conventional engineering materials often sacrifice strength to improve toughness. Researchers hypothesize that nacre's toughness originates within its brick-and-mortar-like microstructure. Under loading, bricks slide relative to each other, propagating inelastic deformation over millimeter length scales. This leads to orders-of-magnitude increase in toughness. Here, we use in situ atomic force microscopy fracture experiments and digital image correlation to quantitatively prove that brick morphology (waviness) leads to transverse dilation and subsequent interfacial hardening during sliding, a previously hypothesized dominant toughening mechanism in nacre. By replicating this mechanism in a scaled-up model synthetic material, we find that it indeed leads to major improvements in energy dissipation. Ultimately, lessons from this investigation may be key to realizing the immense potential of widely pursued nanocomposites. Hierarchical structures are used in nature to yield materials of superior mechanical performance from relatively weak constituents (for example, bone, nacre, wood, spider silk [1] , [2] , [3] , [4] , [5] ). Nacre, the iridescent material found in Abalone shells, exhibits remarkable strength and toughness despite comprising of >95% brittle aragonite ceramic [6] , [7] . With an elegant hierarchical composite structure, nacre is orders of magnitude tougher than pure aragonite [8] , [9] . This extraordinarily tough material is part of a two-layer armour system ( Fig. 1a ) deployed by seashells to protect themselves from predators. A hard calcite outer layer prevents penetration of the shell but is prone to brittle fracture. The tough nacreous inner layer is more compliant and arrests propagating cracks initiating in the brittle outer layer. Understanding the underlying mechanisms by which nature's hierarchical materials achieve improved performance will guide development of novel higher performance composites, and may be a key to achieve full exploitation of the extraordinary properties of nanostructure reinforcement, for example, graphene oxide, carbon nanotubes and clay, in nanocomposites. 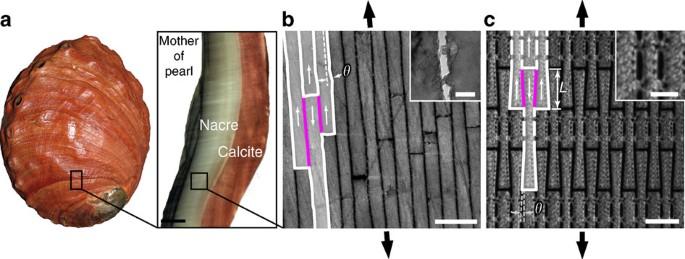Figure 1: Hierarchical structure of natural nacre and bio-inspired composite. (a) Red abalone shell. Inset shows a cross-section cut from the shell. (b) Scanning electron micrograph showing micro/nanostructure of natural nacre. Scale bar, 1 μm. For clarity, a set of tablets is outlined in white. The tablets have two regions, core and overlap17. The overlap region in which relative sliding occurs (arrows indicate direction) is highlighted in magenta. Inset shows a transmission electron micrograph of the inter-tablet bridges23. Scale bar, 100 nm. (c) Artificial composite inspired by nacre, showing dovetailed tablets before polymer infiltration. The length,L, and angle,θ, of the dovetail in the overlap region, are studied parametrically. Scale bar, 5 mm. Inset shows a detail of the inter-tablet bridges. Scale bar, 2 mm. Figure 1: Hierarchical structure of natural nacre and bio-inspired composite. ( a ) Red abalone shell. Inset shows a cross-section cut from the shell. ( b ) Scanning electron micrograph showing micro/nanostructure of natural nacre. Scale bar, 1 μm. For clarity, a set of tablets is outlined in white. The tablets have two regions, core and overlap [17] . The overlap region in which relative sliding occurs (arrows indicate direction) is highlighted in magenta. Inset shows a transmission electron micrograph of the inter-tablet bridges [23] . Scale bar, 100 nm. ( c ) Artificial composite inspired by nacre, showing dovetailed tablets before polymer infiltration. The length, L , and angle, θ , of the dovetail in the overlap region, are studied parametrically. Scale bar, 5 mm. Inset shows a detail of the inter-tablet bridges. Scale bar, 2 mm. Full size image Within nacre's hierarchical structure, toughening mechanisms at multiple length scales have been proposed to contribute to the dramatic improvement in performance. At the microscale, ceramic tablets are stacked like bricks ( Fig. 1b ), with biopolymer lining the interfaces like mortar [10] , [11] . Under loading, these tablets slide relative to each other [12] , [13] , [14] , [15] . It has been proposed that microscale waviness on the surface of the tablets (characterized by angle θ in Fig. 1b ) causes the interface between them to harden as they slide [9] , [15] , [16] , [17] , spreading damage and dissipating energy over large areas to yield superior toughness [9] . A number of nanoscale interlocking mechanisms, activated during sliding, have also been proposed. These include nanoscale asperities on the surface of the tablets that can interlock and increase friction during tablet sliding [13] , mineral bridges ( Fig. 1b inset) that form between adjacent tablets [18] , [19] , [20] , [21] , [22] , [23] , [24] , and unfolding of proteins in the soft interfacial mortar layer [22] , [25] . In addition, unique properties of the tablet themselves were identified such as nanograins [23] , which lead to inelastic deformation and tougher tablets [26] . Although suggested to have a less pronounced effect on the macroscale material behaviour [9] , [16] , [17] , [27] , these nanoscale mechanisms have the potential to contribute to damage spreading. Motivated by the performance of naturally occuring materials, there have been a number of advances in the synthetic materials community designed to mimic the outstanding toughness seen in natural nacre [10] , [28] . Methods to create these materials include large scale layered composites [29] , [30] , ice templation [31] , [32] , freeze casting [33] , layer-by-layer deposition [34] , [35] , [36] , thin film deposition [37] and self-assembly [38] , [39] . Each has produced composites whose performance well exceeds the rule of mixtures. However, in-depth understanding of deformation mechanisms in these materials and how they relate to those observed in nacre remains elusive. Here, we present a comprehensive nanoscale mechanical investigation of the tablet sliding and interfacial hardening mechanisms to which nacre's macroscopic behaviour is attributed. We also discuss their implications to the design of synthetic materials. For the first time, we quantify tablet sliding with nanometre resolution by combining in situ atomic force microscopy (AFM) fracture experiments with kinematic displacement field analysis by digital image correlation (DIC). This analysis highlights the effect of tablet interfacial hardening by revealing transverse expansion at the tablet interfaces (negative Poisson effect), a direct result of compressive stresses generated during tablet sliding-induced interfacial hardening [16] , [17] . On the basis of our investigation of natural nacre, we develop a model synthetic composite specifically incorporating natural nacre's critical tablet sliding and interfacial hardening mechanism (see Supplementary Movie 1 ). This mechanism is implemented in a scaled-up tablet-based design ( Fig. 1c ) by integrating features of the natural nacre structure, including tablets with hardening interfaces (implemented through a dovetail structure) [40] , bridges connecting tablets (designed to constrain transverse expansion of the core region to promote interfacial hardening) and a softer polymer interfacial material to enable tablet sliding. This approach is unique in that, by scaling up, we are able to isolate the interfacial hardening effects generated by the tablet dovetails (analogous to tablet waviness in natural nacre) from smaller scale surface roughness, and thus investigate the mechanistic significance of tablet waviness alone. With this tablet-based synthetic composite, we perform a parametric study to investigate the impact of tablet geometry on the amount of hardening and energy dissipation. Characterization of tablet kinematics using the same DIC process reveals similar degrees of normalized tablet sliding to that of natural nacre. The observation of a ∼ 50% improvement in energy dissipation and strength characteristics of this model composite relative to the bulk tablet material (despite the absence of smaller scale toughening mechanisms) directly verifies the critical role of waviness-induced tablet interfacial hardening. Nanoscale quantification of nacre's toughening mechanisms Pre-notched fracture samples of natural nacre cut from Red Abalone shells were tested in three-point bending [9] and imaged simultaneously with AFM to observe tablet sliding ( Fig. 2 , see also Supplementary Fig. S1 and Methods for details). At each area of interest, a reference image was scanned before loading, followed by incremental loading and imaging until failure. The scanned area was chosen to be within the fracture process zone, roughly 1 mm (ref. 9 ). 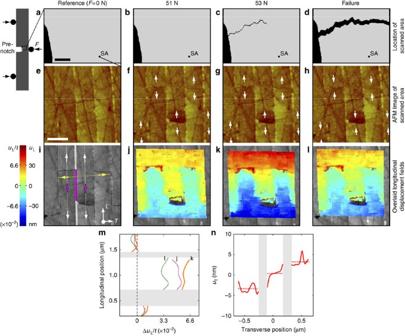Figure 2:In situAFM fracture tests and quantitative analysis of tablet sliding in natural nacre. (a–d) Images showing the position of the scanned area (SA) relative to the pre-notch and propagating crack. Scale bar, 100 μm. (e–h) Series of AFM images of the SA in natural nacre during loading in three-point bending (left ofa). Scale bar, 500 nm, height scale is 50 nm. (e) Reference image captured before loading. (f) The sample has been loaded and tablet sliding is observed (arrows indicate direction as identified in the following DIC analysis). (g) Tablet sliding increases as the crack initiates and propagates towards the SA. (h) Image after sample failure. (i–l) Results of the DIC performed on images (e–h). (i) Reference AFM image (same ase) defining the longitudinal,L, and transverse,T, directions of the tablet coordinate system. For clarity, tablets are outlined in black. The solid white/magenta line highlights the longitudinal interface between two adjacent rows of tables. (j–l) Series of AFM images (f–h) overlaid with DIC longitudinal displacement fieldsuL. Colour scale is displayed both in units of nanometres and normalized by average tablet thicknesst. (m) Plot of relative longitudinal tablet sliding ΔuLin (j–l) along the longitudinal interface between adjacent rows of tablets (solid white/magenta line ini, see alsoSupplementary Informationfor greater detail). The three curves correspond to the three loading states inj–l. (n) Plot of transverse displacement profile,uTat peak load (k) along a line in the transverse direction across three adjacent tablets (dashed yellow line ini, seeSupplementary Informationfor greater detail). Figure 2: In situ AFM fracture tests and quantitative analysis of tablet sliding in natural nacre. ( a – d ) Images showing the position of the scanned area (SA) relative to the pre-notch and propagating crack. Scale bar, 100 μm. ( e – h ) Series of AFM images of the SA in natural nacre during loading in three-point bending (left of a ). Scale bar, 500 nm, height scale is 50 nm. ( e ) Reference image captured before loading. ( f ) The sample has been loaded and tablet sliding is observed (arrows indicate direction as identified in the following DIC analysis). ( g ) Tablet sliding increases as the crack initiates and propagates towards the SA. ( h ) Image after sample failure. ( i – l ) Results of the DIC performed on images ( e – h ). ( i ) Reference AFM image (same as e ) defining the longitudinal, L , and transverse, T , directions of the tablet coordinate system. For clarity, tablets are outlined in black. The solid white/magenta line highlights the longitudinal interface between two adjacent rows of tables. ( j – l ) Series of AFM images ( f – h ) overlaid with DIC longitudinal displacement fields u L . Colour scale is displayed both in units of nanometres and normalized by average tablet thickness t . ( m ) Plot of relative longitudinal tablet sliding Δ u L in ( j – l ) along the longitudinal interface between adjacent rows of tablets (solid white/magenta line in i , see also Supplementary Information for greater detail). The three curves correspond to the three loading states in j – l . ( n ) Plot of transverse displacement profile, u T at peak load ( k ) along a line in the transverse direction across three adjacent tablets (dashed yellow line in i , see Supplementary Information for greater detail). Full size image Figure 2e–h shows a series of AFM images captured in the scanned area during loading and after sample failure. This is a representative case selected from a number of tests showing similar results (see Supplementary Information and Methods for more results and discussion of the behaviour at different scales and at different locations relative to the propagating crack). Imaging throughout the incremental loading process allowed characterization of material deformation before, during and after crack propagation. Post-processing of the images using DIC enabled (see Supplementary Fig. S2 ), for the first time, quantification of tablet sliding, as well as identification of transverse dilation of tablets during crack propagation, all with sub-nanometer resolution ( ∼ 1/10 pixel [41] or 0.4 nm). To quantify the observed sliding, post-processing was performed on the series of AFM images using Kelkins DIC package (see Supplementary Methods ). Figure 2i–l shows the same series of AFM images overlaid with the computed longitudinal component of the displacement field, u L , that is, aligned with the long axis of the tablets. As the crack initiates and approaches the scanned area ( Fig. 2j,k ), progressive sliding is seen through increasing colour intensity in the DIC displacement fields. After the crack passes above the scanned area ( Fig. 2l ), a partial reversal of the displacement field occurs, resulting in partial closure of the gap between tablet ends. The corresponding relative sliding at the interface between two rows of adjacent tablets is plotted in Figure 2m . This is computed by taking the longitudinal displacement profile along the centrelines of two adjacent tablets (dashed white lines in Fig. 2i ) and projecting their difference onto the interface between them (solid white/magenta line in Fig. 2i , see Supplementary Methods ). In Figure 2j–l , rigid body displacements were removed to highlight the relative sliding of the overlapping tablets. This corresponds to the sliding of 'stacks' or 'columns' of tablets as identified by Gilbert et al . [42] As expected, the graph shows a discontinuous jump in relative displacement occurring in the overlap region between adjacent tablets (magenta segment of interfacial line). The fact that there is significant relative sliding only within the overlap region intuitively suggests that any sliding-induced interfacial hardening mechanism will be activated only within this overlap region. Within the core region, the tablets deform elastically with near-zero relative motion. DIC also revealed nanoscale dilation of the tablets in the direction transverse to tablet sliding. Figure 2n shows the transverse displacement profile, u T , along a line across three adjacent tablets (dashed yellow line Fig. 2i ). Global rigid body motion was corrected such that the negative average displacement of the left-most tablet indicates that it is moving to the left, whereas the positive displacement of the right-most tablet indicates that it is moving to the right, all with respect to the central tablet (that is, an overall transverse expansion). The grey bands in Figure 2m,n correspond to the biopolymer-filled interfaces at the ends and in between tablets. Because the thickness of these interfaces is small relative to the imaging resolution, they were not well resolved and thus excluded from the analysis. The transverse displacements, whose evolution correlates to that of the longitudinal sliding, provides powerful confirmation of the critical role of tablet waviness and interfacial hardening in nacre's toughening. Because of their inherent, and initially commensurate, waviness ( Fig. 1b ), relative longitudinal sliding induces transverse compressive stresses and displacement as one wavy tablet surface slides over the wavy surface of the adjacent tablet. This dilation effect was observed consistently at different regions relative to the propagating crack and in multiple samples (see also Supplementary Figs S3 and S4 , and Methods). 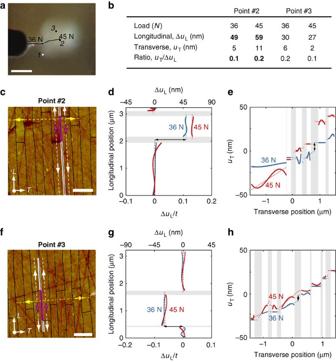Figure 3: Comparing longitudinal and transverse tablet displacements at different regions relative to the crack. (a) Image showing the position of the scanned areas relative to the propagating crack and the surrounding inelastic zone (whitish appearance). The location of the crack tip at different loads is indicated. Points 2 and 3 were taken on the same sample in a single test. Point 1 indicates the relative position of the scanned area from a different test shown inFigure 2. Because these points were taken on different samples, a representative image9is used here. Scale bar, 500 μm. (b) Table summarizing the applied load, longitudinal sliding and transverse displacement across the interfaces taken from (d,e) and (g,h). The transverse displacement was taken as the average jump inuTacross each interface between tablets (grey bands ine, see alsoSupplementary Information). (c–e) Results from point 2. (c) Reference image captured before loading. For clarity, tablets are outlined in black. The solid white/magenta line highlights the longitudinal interface between two adjacent rows of tables. Scale bar, 1 μm. (d) Plot of relative longitudinal tablet sliding ΔuLin (c) along the longitudinal interface between adjacent rows of tablets (solid white/magenta line inc, see alsoSupplementary Information). The two curves correspond to the two different loading states. (e) Plot of transverse displacement profile,uT, at the two loading states along a line in the transverse direction across three adjacent tablets (dashed yellow line inc, see alsoSupplementary Information). (f–h) Results from point 3 showing the same analysis asc–e. Figure 3 shows the longitudinal and transverse tablet displacements at different locations relative to the crack. Close to the crack (point 2, Fig. 3c–e ) the longitudinal sliding and corresponding transverse dilation are more pronounced. In fact, the progressive hardening becomes directly evident at point 2. As the load increases from 36 to 45 N and the crack propagates towards the scanned area ( Fig. 3a ), the relative longitudinal sliding and transverse dilation increase as expected ( Fig. 3b,d,e ). Moreover, the ratio of the longitudinal to transverse displacement also increases ( Fig. 3b,e ), which is indicative of increasing transverse compressive stresses acting to harden the interface and reduce longitudinal sliding. At point 3, which is further from the crack than point 2 ( Fig. 3a ), lesser degrees of tablet sliding are observed ( Fig. 3b,g,h ). The tip of the crack passes point 3 as the load increases from 36 to 45 N. Thus, a slight relaxation in longitudinal and transverse tablet displacements is observed. Figure 3: Comparing longitudinal and transverse tablet displacements at different regions relative to the crack. ( a ) Image showing the position of the scanned areas relative to the propagating crack and the surrounding inelastic zone (whitish appearance). The location of the crack tip at different loads is indicated. Points 2 and 3 were taken on the same sample in a single test. Point 1 indicates the relative position of the scanned area from a different test shown in Figure 2 . Because these points were taken on different samples, a representative image [9] is used here. Scale bar, 500 μm. ( b ) Table summarizing the applied load, longitudinal sliding and transverse displacement across the interfaces taken from ( d , e ) and ( g , h ). The transverse displacement was taken as the average jump in u T across each interface between tablets (grey bands in e , see also Supplementary Information ). ( c – e ) Results from point 2. ( c ) Reference image captured before loading. For clarity, tablets are outlined in black. The solid white/magenta line highlights the longitudinal interface between two adjacent rows of tables. Scale bar, 1 μm. ( d ) Plot of relative longitudinal tablet sliding Δ u L in ( c ) along the longitudinal interface between adjacent rows of tablets (solid white/magenta line in c , see also Supplementary Information ). The two curves correspond to the two different loading states. ( e ) Plot of transverse displacement profile, u T , at the two loading states along a line in the transverse direction across three adjacent tablets (dashed yellow line in c , see also Supplementary Information ). ( f – h ) Results from point 3 showing the same analysis as c – e . Full size image Dilation has also been observed at larger scales in tensile and shear strain fields obtained by means of optical DIC across areas of 100 s of microns. In tension, dilation was identified following an initial transverse contraction due to the Poisson effect [9] , [17] . The nanoscale investigation, herein, enables identification of this behaviour on a local tablet level, thus confirming the occurrence of interfacial hardening induced by relative sliding of wavy interfaces. Translating nacre's toughening mechanisms to a bio-inspired model composite Applying the lessons from natural nacre, we designed a hierarchical synthetic material (artificial nacre) that not only increases strength to failure, but also dissipates more energy by increasing the strain to failure. The tablet-based structure ( Fig. 1c , and Supplementary Figs S5 and S6 ) of this composite incorporates critical features from its natural inspiration, namely: tablets whose interface hardens during sliding, solid bridges between tablets and a soft epoxy interfacial material to facilitate sliding. For this mesoscale material, we chose to implement tablet interfacial hardening via a dovetailed tablet structure, rather than the more random waviness observed in natural nacre. The tablets were made from acrylonitrile butadiene styrene (ABS) plastic through rapid prototyping (fused deposition moulding). The interfacial gap between tablets was then infiltrated with Dow Chemical flexibilized epoxy (see Methods ). The artificial nacre samples were tested in tension to assess their performance and deformation mechanisms as they compare with natural nacre. A subsequent parametric study of the tablet geometry enabled design optimization and further confirmed the critical role of interfacial hardening during tablet sliding. To determine the optimal tablet geometry that would tolerate high stresses and strains while maximizing the dissipated energy, we fabricated and tested artificial samples with varying dovetail angles θ and dovetail overlap lengths L ( Figs 1c and 4a–c ). The same DIC technique used for natural nacre was applied to quantify tablet sliding in the artificial nacre; this time on images acquired optically with a resolution of 45 μm per pixel ( Fig. 4d–g , Supplementary Methods ). 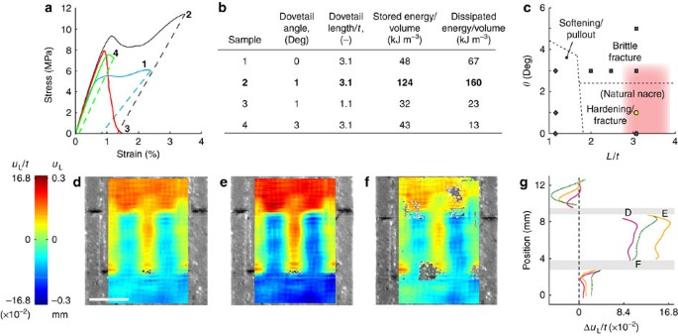Figure 4: Assessing ABS-epoxy nacre-inspired composite performance. (a) Engineering stress–strain curves for artificial nacre samples with varying dovetail length and angle (labelled by sample number as listed inb). SeeSupplementary Informationfor unloading behaviour and repeatability of the constitutive behaviour. (b) Table showing normalized stored and dissipated energies for samples of varying tablet geometry. Dovetail lengths (L=2.1 and 5.7 mm) have been normalized by tablet thickness (t=1.85 mm). (c) Map of identified failure modes as they relate to the dovetail angleθand lengthL(normalized by tablet thicknesst). Sample #2, which exhibits the greatest energy storage and dissipation per unit volume, see (b), is indicated with a yellow-filled circle. The structure of natural nacre falls within the red area (seeSupplementary Information). (d–f) Series of optical images of artificial composite sample #2 overlaid with DIC longitudinal displacement fieldsuLshowing progressive tablet sliding (d,e) and subsequent partial relaxation (f) after failure. Scale bar, 4 mm. Colour scale is displayed both in units of millimeters and normalized by average tablet thicknesst. (g) Plot of relative longitudinal tablet sliding ind–falong the longitudinal interface between adjacent tablets. The three curves correspond to the three loading steps ind–f. Figure 4: Assessing ABS-epoxy nacre-inspired composite performance. ( a ) Engineering stress–strain curves for artificial nacre samples with varying dovetail length and angle (labelled by sample number as listed in b ). See Supplementary Information for unloading behaviour and repeatability of the constitutive behaviour. ( b ) Table showing normalized stored and dissipated energies for samples of varying tablet geometry. Dovetail lengths ( L =2.1 and 5.7 mm) have been normalized by tablet thickness ( t =1.85 mm). ( c ) Map of identified failure modes as they relate to the dovetail angle θ and length L (normalized by tablet thickness t ). Sample #2, which exhibits the greatest energy storage and dissipation per unit volume, see ( b ), is indicated with a yellow-filled circle. The structure of natural nacre falls within the red area (see Supplementary Information ). ( d – f ) Series of optical images of artificial composite sample #2 overlaid with DIC longitudinal displacement fields u L showing progressive tablet sliding ( d , e ) and subsequent partial relaxation ( f ) after failure. Scale bar, 4 mm. Colour scale is displayed both in units of millimeters and normalized by average tablet thickness t . ( g ) Plot of relative longitudinal tablet sliding in d – f along the longitudinal interface between adjacent tablets. The three curves correspond to the three loading steps in d – f . Full size image Supplementary Movie 1 shows the progression of sliding during loading. In general, we see that tablet sliding initiates at a certain strain, and propagates uniformly throughout the sample. With no dovetail ( θ =0), negligible hardening after yielding and relatively low peak stress was observed ( Fig. 4a-1 ) because of the lack of an interfacial hardening mechanism. With a dovetail angle, θ , of 1° (and maintaining the same dovetail overlap length), we measured the greatest degree of sliding, the highest stress and strain before failure, and the greatest energy dissipation per unit volume, 160 kJ m −3 ( Fig. 4a-2,b and Supplementary Figs S7–S10 ). This is an improvement of more than 100% over the 0° sample and ∼ 50% over the bulk ABS tablet material, which alone dissipated 110 kJ m −3 . Here, the interfacial hardening effect was clearly present in the stress–strain response, which exhibited significant hardening following the onset of yielding (sliding). This high rate of hardening, which is at least one order greater than that observed in the 0° sample, is important in delaying the onset of necking instabilities. The longitudinal DIC displacement fields, u L , for this sample are shown in Figure 4d–g and Supplementary Figure S9 , with a precision of 20 μm. Looking at the relative longitudinal sliding ( Fig. 4g ), we see that it is very similar to that of natural nacre ( Fig. 2m ). As before, we see sliding only in the overlap region between tablets, which increases with progressive loading, followed by partial relaxation on failure. With shorter dovetail lengths, softening and tablet pullout occurred at lower stresses and strains ( Fig. 4a-3 ), resulting in dramatically less energy dissipation. For larger dovetail angles, the interfacial hardening strength was greater than that of the tablets themselves, and localized brittle tablet failure was observed ( Fig. 4a-4 ). Figure 4c shows a parametric map of failure modes for the artificial nacre as a function of tablet geometry. Interestingly, the tablet geometry of the artificial sample exhibiting the greatest energy dissipation (sample #2, Fig. 4b ) falls directly within the range of tablet geometries found in natural nacre, accounting for statistical variations, when they are overlaid on the same map ( Fig. 4c ). In addition, the hardening/fracture failure mechanism observed in the optimal sample is similar to that observed in natural nacre ( Supplementary Information ). These results provide additional evidence that sliding-induced tablet interfacial hardening is the primary mechanism leading to an increase in both strength and ductility, similar to natural nacre. Moreover, greater distribution of sliding across the material translates to an increase in dissipated energy and toughening, which contributes to natural nacre's outstanding crack arresting performance. Similar to natural nacre, we also measured transverse dilation in the artificial material. However, because the tablets are made from relatively soft ABS compared with stiff ceramic, they develop a transverse compressive strain also present in the epoxy filler material, making transverse displacement differences across tablets less pronounced. The primary finding of this paper is that sliding of microscale wavy tablets relative to each other results in dilation-induced hardening of the interface between tablets, which results in an increase in toughness. The measurement of a transverse expansion (negative Poisson's ratio) at the nanoscale is a direct result of the transverse compressive stresses generated by this sliding-induced interfacial hardening, and thus confirms the activation of this toughening mechanism. We have shown that the degree of tablet displacement (longitudinal sliding and transverse dilation) is dependent on the location relative to the crack tip. Farther from the crack tip we see less pronounced transverse dilation and tablet sliding. However, close to the crack (position 2 in Fig. 3 ), we see that as the load increases, the ratio of tablet sliding to transverse dilation increases, which greatly supports the notion of interfacial hardening during tablet sliding. This increasing transverse compression acts to increase load transfer between tablets, reducing relative sliding. Translation of this interfacial hardening mechanism to a scaled-up (approximately four orders of magnitude), bio-inspired model composite exhibiting significant improvement in energy dissipation shows the effectiveness of such a mechanism, even in the absence of smaller asperities. This continued demonstration, in spite of the drastic scaling, speaks to the elegance of natural designs and the identification of a key mechanism leading to damage spreading. Using DIC we confirmed that tablet sliding in the overlap region, for the artificial nacre-like material, was qualitatively similar to that of natural nacre. Through a parametric study of the ABS-epoxy composite, we found that an intermediate dovetail angle of 1° and overlap length of three times the tablet thickness provided the optimal level of interfacial hardening to maximize stress, strain and energy dissipation. Here, it is important to note that this particular optimal geometry is specific to this ABS-epoxy material system and length scale. Through the use of more brittle tablet materials (different from ABS), similar or greater levels of improvement in energy dissipation should be possible without sacrificing strength. Because of the observed increase in strength and strain to failure of the optimized artificial composite ( Fig. 4a-2 ), we conclude that tablet sliding and interfacial hardening can have a significant impact on toughening in nacre (whose ductility has been widely reported [7] , [9] , [13] , [17] ). Looking at the failure mode map ( Fig. 4c ), we observed that the highest performing artificial nacre tablet geometry corresponded directly to the structure of natural nacre, suggesting that our bio-inspired parametric study arrived at a similarly optimized design to that of Nature's evolution process. Ultimately, a twofold improvement of dissipated energy was achieved in this composite compared with the bulk material. The experiments reported in this work were motivated by a need for a deeper understanding of nacre's hierarchical structure in an effort to create synthetic composites that leverage similar mechanisms. As such, the reported results have strong implications for the biomimetic and composites fields. To place these findings in the context of the highly active field of nanocomposites, we briefly note how these lessons can be applied to widely pursued graphene, graphene oxide, nanotube and clay composites. The potential of these constituents in very high volume fractions is evident from their outstanding mechanical properties (for example, carbon nanotubes exhibit tera -Pascal modulus and strengths in excess of 100 GPa (ref. 43 )). The present study shows that creating an interface, which hardens during relative sliding of reinforcing elements, is essential to confer defect and stress-induced damage tolerance to the material. Although challenging at the nanoscale, modifications can be made to improve lateral interaction (similar to waviness-induced interfacial hardening) between reinforcement elements. For example, molecular kinks or bumps can be introduced to graphene sheets through functionalization [44] . These may act similar to the waviness or asperities on the surface of nacre tablets. Chemical bonds (for example, covalent crosslinks) could serve a similar purpose as the mineral bridges between nacre tablets, constraining transverse expansion to promote interfacial hardening. Interfacial friction between carbon nanotubes within bundles can also be enhanced by using pressure to collapse the nanotubes [45] . As such, the majority of the design space for nanocomposites encompasses the nature of the interfacial material and its interaction with the reinforcing constituents. In keeping with the lessons learned from nacre, the interfacial molecules, their length and their interaction with the reinforcement (chemical bond type and density) should be chosen not to simply be as strong as possible (as it is commonly believed), but rather to allow controlled sliding by incorporating hardening mechanisms that are activated during shear interactions. Such a mechanism would ensure diffusive inelastic shearing, as observed in nacre, and high toughness. Within this scope, auxetic molecules, which exhibit a negative Poisson's ratio at the molecular level, are a promising class of materials for the matrix component of nanocomposites. As these molecules are stretched, they expand in the transverse direction, generating compressive stresses similar to the dovetails of the artificial nacre structure [46] , [47] , [48] , [49] , [50] . Incorporating this type of molecule in the design of nanocomposites remains a wide-open opportunity. Achieving interfacial hardening mechanisms, using auxetic molecules, will require selection of compatible surface functional groups to serve as anchors between these molecules and the stiff constituents. Accordingly, the design space ( Fig. 5 ) will include type (for example, carboxyl, hydroxyl, epoxy) and degree of surface functionalization (density of anchors, for example, carbon to oxygen ratio in graphene oxide [51] , [52] ). 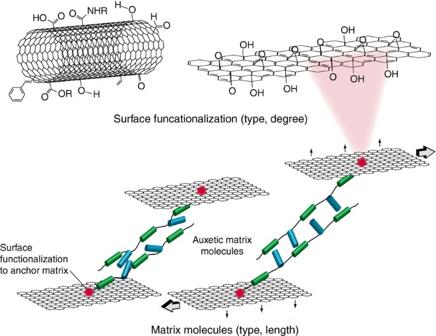Figure 5: Design space for emerging nanocomposites. Instead of constituent geometry, interface chemistry is used to control lateral interactions. In this context, auxetic molecules are envisioned as candidates to achieve controlled interfacial hardening. Figure 5: Design space for emerging nanocomposites. Instead of constituent geometry, interface chemistry is used to control lateral interactions. In this context, auxetic molecules are envisioned as candidates to achieve controlled interfacial hardening. Full size image In summary, lessons learned from nacre may provide key ideas to realize nanocomposites with high resilience (that is, defect tolerance). Given that atomic and other defects are ubiquitous in materials, conferring them with tolerance to such defects is a paradigm shift in nanocomposite design that requires more vigorous pursuit. The incorporation of progressively hardening interfaces may offer one such path to enable performance scaling and the achievement of ultra strong and tough composites. Fracture experiments on natural nacre Nacre samples were cut from large Abalone shells for three-point-bend testing in accordance with American Society for Testing and Materials (ASTM) standard E-1820. Supplementary Figure S1 shows a schematic of the sample preparation process. An Accutom saw (Struers) with a 330 CA blade (Struers) was used to cut oversized samples from the full shell. A thin 0.012 inch diamond blade (Primecut blade, Crystalite Corporation) was then used to cut the final dimensions and pre-notch of the specimen. Finally, Buehler water-based diamond particle polishing solutions (Buehler) were used to polish the samples in stages from 9 μm down to 0.5 μm particle sizes on a Texmet polishing cloth (Buehler). After preparation, samples were tested in three-point-bending in situ a Veeco Instruments DI 3100 AFM (Veeco). A displacement-controlled miniature tensile testing machine (Ernest F. Fullam, Inc.) was mounted on the AFM stage, enabling simultaneous loading and imaging. A linear variable displacement transducer and 100 pound load cell (Honeywell Sensotec) integrated in the Fullam machine enabled measurement of crosshead displacement and load during testing. To minimize the effects of thermal drift, the Fullam system was mounted in the AFM at least 12 h before use to allow the temperatures of the systems to equilibrate. To further reduce thermal effects, the AFM and Fullam stage were turned on and allowed to run for several hours before conducting each test to ensure they reached a stable operating temperature (the temperature within the AFM chamber was observed to rise ∼ 1 °C within the first 30 min of running the equipment and then stabilize). All samples were imaged in tapping mode at a resolution of 512 samples (pixels) per line, and 512 lines per image. Before loading, an area of interest around the pre-notch was imaged as a reference for the DIC analysis. To avoid the influence of traction-free boundary conditions, we chose a region not too close to the crack. The sample was then incrementally loaded and imaged repeatedly until failure in the same area of interest. With these images we were able to capture nacre's material response before, during and after crack propagation. The high-resolution AFM images were then analysed through DIC to quantify the amount of tablet sliding. Details of the DIC technique are discussed in Supplementary Methods . Investigating tablet sliding and transverse expansion at different locations relative to the crack Investigating the displacement of tablets at various distances from the crack path is critical to building a comprehensive understanding of the toughening mechanisms in nacre. Previous work by Barthelat, et al . applied DIC techniques to investigate displacements at larger fields of view (100 s of microns [9] , [17] ). In this work, we focused on the micro- and nanoscale (single tablet scale) mechanisms occurring at different regions relative to the propagating crack, which contribute to this large-field behaviour. As described in refs 13 and 9 , a white region can be observed in regions of stress where inelastic deformation (tablet sliding) has occurred. As the loading increases, this inelastic zone expands and then begins to propagate forward as the crack propagates. As expected, the intensity of this whiteness, which is proportional to the degree of tablet sliding, is greatest at the crack and decays going away from it. Thus, the intensity of this white region can be used to identify distinct regions of differing degrees of inelastic deformation to investigate relative to the crack. Figure 3a in the manuscript shows the inelastic zone during crack propagation and the position of the reported results within this zone. Using the same DIC technique (see Supplementary Methods for detailed description), we calculated the longitudinal sliding and transverse dilation of tablets at points 2 and 3 from Figure 3a . This enabled comparison of tablet displacement behaviour at different regions relative to the crack. Supplementary Figures S3 and S4 show the longitudinal displacement fields, longitudinal tablet sliding and transverse dilation of the tablets for points 2 and 3, respectively. In general, greater degrees of longitudinal sliding and transverse dilation are observed closer to the crack (point 2 versus point 3). At point 2 ( Supplementary Fig. S3 ), the crack approaches the scanned area as the load increases from 36 to 45 N ( Fig. 3a ). Thus, the tablet displacements increase between the two loading steps. At point 3 ( Supplementary Fig. S4 ), the crack passes by the scanned area as the load increases from 36 to 45 N ( Fig. 3a ). Thus, the tablet displacements relax slightly between the 36 and 45 N load steps. This decreasing degree of tablet sliding farther from the crack is representative of damage spreading and energy dissipation. Furthermore, at point 2, an increase in the ratio of transverse to longitudinal tablet displacement is observed with increasing longitudinal sliding (see summary in Fig. 3b ). This observation speaks to the activity of the interfacial hardening mechanism, as the increasing rate of transverse expansion relative to longitudinal sliding is a direct result of transverse compressive stresses building in the tablets as they slide. These stresses have been predicted previously through finite element simulations [17] . Artificial nacre design and fabrication The artificial nacre samples were fabricated using ABS through a fused deposition modelling (FDM) rapid prototyping technique (FDM Titan, Stratasys) at General Motors R&D Laboratories. A unit cell of the fabricated sample is shown in the inset of Supplementary Figure S6 , as well as a schematic of the full sample. This design exhibits nacre's main sliding-induced toughening mechanism. Rather than using complex wavy tablets as found in natural nacre, interfacial hardening is created through a dovetailed tablet geometry (dovetail angle θ and dovetail length L ). To create a columnar structure similar to nacre, long tablets are arranged with shorter tablets mimicking the core and overlap regions in nacre ( Supplementary Fig. S6 ). The inter-tablet mineral bridges found in natural nacre are also replicated here ( b in Supplementary Fig. S6 ). To determine the material properties of the bulk ABS material used for the tablets, dogbone samples using ASTM standard D638-08 were tested in tension. Images during the test were acquired optically (rather than by AFM as for the natural nacre) with a Navitar macro lens and a CCD camera giving a typical resolution of 45 μm per pixel. The same DIC software previously mentioned accurately calculated the strain in the gage region. Supplementary Table S1 summarizes the ultimate strength, Young's modulus and plastic strain to failure. On the basis of these results, we then selected an infiltration material to fill the interfaces knowing that it must have relatively low strength but high elongation to failure to allow tablet sliding. Accordingly, we chose a DOW Chemical flexibilized epoxy, specifically a 50–50% mixture of D.E.R. 732 and D.E.R. 331 with the addition of D.E.H. 24 hardener. Using the same ASTM standards, dogbone samples of the epoxy were made and tested. Again, DIC confirmed the amount of strain in the gage region of the sample. Properties for this material are shown in Supplementary Table S1 . The ABS pre-forms from Supplementary Figure S6 were infiltrated with the epoxy and cured for 1 week. After curing, the samples were machined to remove excess epoxy by milling. Samples were tested until failure using a MTS Syntec 20/G tensile testing machine at a constant crosshead displacement rate of 0.2 mm min −1 . A parametric study varying dovetail angle ( θ : 0–5°) and dovetail length ( L : 2.12–5.7 mm) verified an optimal design with the greatest strength and elongation to failure (over 35 tested samples). Performance was compared based on the amount of energy stored and dissipated per unit volume. These energies were calculated from the area beneath the stress–strain curve as shown in Supplementary Figure S7 . A representative set of these results are reported in Figure 4 of the manuscript. Supplementary Figure S8 shows the results of multiple tests for the various geometries reported in Figure 4 . Although the stress and strain at failure for a given sample geometry varies to some degree (likely due to variations in defects arising from the infiltration), the characteristic behaviour (for example, softening and subsequent hardening) remains consistent. How to cite this article: Espinosa, H. D. et al . Tablet-level origin of toughening in abalone shells and translation to synthetic composite materials. Nat. Commun. 2:173 doi: 10.1038/ncomms1172 (2011).